Soft epitaxy of nanocrystal superlattices Epitaxial heterostructures with precise registry between crystal layers play a key role in electronics and optoelectronics. In a close analogy, performance of nanocrystal (NC) based devices depends on the perfection of interfaces formed between NC layers. Here we systematically study the epitaxial growth of NC layers for the first time to enable the fabrication of coherent NC layers. NC epitaxy reveals an exceptional strain tolerance. It follows a universal island size scaling behaviour and shows a strain-driven transition from layer-by-layer to Stranski–Krastanov growth with non-trivial island height statistics. Kinetic bottlenecks play an important role in NC epitaxy, especially in the transition from sub-monolayer to multilayer coverage and the epitaxy of NCs with anisotropic shape. These findings provide a foundation for the rational design of epitaxial structures in a fundamentally and practically important size regime between atomic and microscopic systems. Traditional semiconductor technology utilizes the epitaxy process to build perfect interfaces where the atomic lattice of a crystalline substrate is used to guide the growth of a new material, an epitaxial adlayer [1] . The significant body of knowledge developed about atomic and molecular epitaxy [2] , [3] , [4] has been recently complemented by studies of micron-size colloidal particles tracked by optical microscopy [5] , [6] , [7] . In the present study, we examine the epitaxial growth of superlattices composed of sub-10 nm metal and semiconductor nanocrystals (NCs). Colloidal NCs have the potential to replace atoms as the basic building blocks of modern materials, owing to their tunable properties and interactions and ability to self-assemble into macroscopic ordered superstructures [8] , [9] , [10] , [11] . Recent fundamental studies on energy [12] , charge [13] and heat [14] transport have provided the foundation for the rational design of NC-based electronic devices [13] , [15] , [16] . As in the case of traditional semiconductor devices, the formation of epitaxial interfaces between NC superlattices is an essential prerequisite for efficient NC devices. For example, NC solar cells and light detectors require stacked NC layers with n- and p-type conductivity for efficient separation of charge carriers [16] . In addition to their technological potential, colloidal NCs are a convenient model system. Their size can be precisely tuned [8] , enabling us to isolate the effect of lattice misfit. NCs can also adopt various shapes [9] and spontaneously self-assemble into higher-order structures, including binary and ternary superlattices [10] , [11] . This allows for the exploration of epitaxy in complex systems not accessible with atoms or micron-size particles. Our work also serves as an example for epitaxy driven by ‘soft’ inter-NC forces. Understanding the behaviour of ‘soft’ materials in the nanometer size regime is of fundamental importance because many chemical and biological species (macromolecules, nanostructures, proteins, viruses and so on.) naturally belong to it. Epitaxial assembly of NCs We study the epitaxy of Au NCs ( Fig. 1 ) on the surface of monolayers of PbS NCs that are used as the substrate. An example of a PbS NC monolayer self-assembled at the air/water interface and transferred to a polished silicon wafer is shown in Fig. 2a (refs 17 , 18 ). The PbS NC monolayers exhibit strong van der Waals adhesion to the silicon substrate, and after drying at ambient conditions for several days, show no tendency to dissolve or swell when immersed in toluene or hexane ( Supplementary Fig. 1 and Supplementary Note 1 ). Scanning electron microscopy (SEM) and atomic force microscopy (AFM) images of NC monolayers reveal long-range hexagonal order with periodic height variations ( Fig. 2a ). The degree of hexagonal order is evaluated by the determination of individual NC positions and construction of Voronoi tessellations [18] , [19] , which are colour coded by the orientation of the ‘bonds’ connecting centres of neighbouring NCs, as indicated in the bond angle plot ( Fig. 2a , upper inset). The distribution of bond lengths ( l ) is represented by histograms of the Voronoi cell (here equivalent to the Wigner–Seitz cell) area A= √3 l 2 /2 ( Fig. 2c ) corresponding to <5% dispersion of NC sizes. 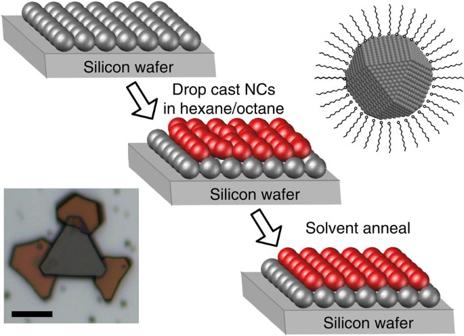Figure 1: Scheme of the epitaxial assembly process. Self-assembled NC monolayers serve as substrates to control the organization of deposited NCs. NCs in a 9:1 hexane/octane solution are drop cast onto NC monolayers and assemble as the solvent evaporates. After the initial deposition, the assemblies are solvent annealed in toluene vapour at 40 °C to improve organization of the epitaxial adlayer. Upper inset: sketch of a nanocrystal with organic capping ligands. Lower inset: optical image of a heterostructure supercrystal composed of 3.2 nm CdSe (orange crystals) and 7.3 nm PbS NCs (grey-centred crystal). Scale bar, 10 μm. Figure 1: Scheme of the epitaxial assembly process. Self-assembled NC monolayers serve as substrates to control the organization of deposited NCs. NCs in a 9:1 hexane/octane solution are drop cast onto NC monolayers and assemble as the solvent evaporates. After the initial deposition, the assemblies are solvent annealed in toluene vapour at 40 °C to improve organization of the epitaxial adlayer. Upper inset: sketch of a nanocrystal with organic capping ligands. Lower inset: optical image of a heterostructure supercrystal composed of 3.2 nm CdSe (orange crystals) and 7.3 nm PbS NCs (grey-centred crystal). Scale bar, 10 μm. 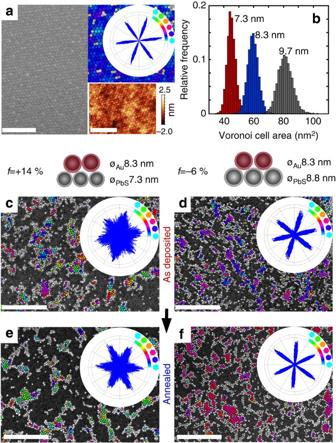Figure 2: Epitaxial assembly of nanocrystals. (a) SEM image of a 9.7 nm PbS NC monolayer. Upper inset: blue hexagons are Voronoi cells superimposed over NCs. The colour coding shows the orientation of the Voronoi cells which is also represented by the bond angle plot. Lower inset: AFM image of an 8.8 nm PbS NC monolayer. Scale bars, 100 nm. (b) Distribution of Voronoi cell areas for monolayers composed of different diameter PbS NCs. (c–f) SEM images and bond angle plots (insets) of Au NCs assembled on PbS NC monolayers before (c,d) and after (e,f) solvent annealing at different lattice misfits,f=(dAu−dPbS)/dPbS,(c,e)f=+14% and (d,f)f=−6%, (schemes). Voronoi cells superimposed over Au NCs with hexagonal symmetry are colour coded according to their orientation with respect to the underlying PbS NC lattice. Extended area images ofc,eandd,fare given inSupplementary Figs 5and6, respectively. Scale bars inc–f, 200 nm. Full size image Figure 2: Epitaxial assembly of nanocrystals. ( a ) SEM image of a 9.7 nm PbS NC monolayer. Upper inset: blue hexagons are Voronoi cells superimposed over NCs. The colour coding shows the orientation of the Voronoi cells which is also represented by the bond angle plot. Lower inset: AFM image of an 8.8 nm PbS NC monolayer. Scale bars, 100 nm. ( b ) Distribution of Voronoi cell areas for monolayers composed of different diameter PbS NCs. ( c – f ) SEM images and bond angle plots (insets) of Au NCs assembled on PbS NC monolayers before ( c , d ) and after ( e , f ) solvent annealing at different lattice misfits, f =( d Au − d PbS )/ d PbS, ( c , e ) f =+14% and ( d , f ) f =−6%, (schemes). Voronoi cells superimposed over Au NCs with hexagonal symmetry are colour coded according to their orientation with respect to the underlying PbS NC lattice. Extended area images of c , e and d , f are given in Supplementary Figs 5 and 6 , respectively. Scale bars in c – f , 200 nm. Full size image To study the formation of an epitaxial interface between superlattices made of different NCs, such as those shown in the bottom-left inset of Fig. 1 and Supplementary Figs 2 and 3 , colloidal Au NCs are deposited on PbS NC monolayers and the carrier solvent (9:1 hexane:octane by volume) is allowed to evaporate ( Fig. 1 ). Analogous to atomic epitaxial growth, the periodic surface potentials defined by PbS NC monolayers guide the self-assembly of Au NC adlayers ( Supplementary Fig. 4 ). The coverage θ , defined as the number of deposited NCs per each available lattice site in the PbS NC substrate [2] , [3] , is varied from sub-monolayer to multilayer coverage. We change the size of PbS NCs in the substrate layer ( Fig. 2b ), while keeping the size of Au NCs constant to cover a wide range of lattice misfits without changing the chemical nature of the NCs ( Supplementary Table 1 and Supplementary Note 2 ). The lattice misfit is defined as f=(b−a)/a , where a and b are the centre-to-centre distances of NCs in unstrained substrate and adlayer lattices, respectively. The misfit is positive (compressive) when b>a and negative (tensile) when b<a (ref 2 ). The contrast in brightness between Au and PbS NCs in SEM images allows for selective analysis of NCs in either the substrate or adlayer [18] . Tracked SEM images of assemblies formed by depositing 8.3 nm Au NCs over 7.3 nm ( f =+14%) and 8.8 nm ( f =−6%) PbS NC monolayers are shown in Fig. 2c,d , respectively, where the samples have similar island sizes. The degree of adlayer alignment can be evaluated by the colour uniformity of the Voronoi cells and the sharpness of the bond angle plots. Fast evaporation of the carrier solvent results in poor alignment of the Au NC adlayer with the PbS NC substrate for f =+14%, while the alignment significantly improves for f =−6%. To relax the system towards an energetically stable configuration, we anneal samples in toluene vapour at 40 °C, typically for 2 h (ref. 18 ). The quality of the adlayer alignment significantly improves after solvent annealing, as indicated by the increased sharpness of the bond angle plots ( Fig. 2e,f ). Solvent annealing also reduces the dispersion in Voronoi cell areas down to that of the underlying PbS NC monolayer ( Fig. 3a ). The efficient strain relaxation is also illustrated through the reduction of both isotropic and shear strain in the Au NC adlayer after solvent annealing ( Fig. 3b,c , respectively) [18] . Annealing for different lengths of time (15 min–18 h) shows that 60 min is sufficient for strain relaxation and attaining a stable state for NC adlayer. At this point, no further reductions in the bond angle dispersion are observed as the system has approached an equilibrium state ( Supplementary Fig. 7 and Supplementary Table 2 ). In general, we observe better alignment for f ≤0 compared with f >0, both before and after solvent annealing, which is consistent with the strong anharmonicity of inter-NC potentials where steric repulsion is steeper than van der Waals attraction [2] . 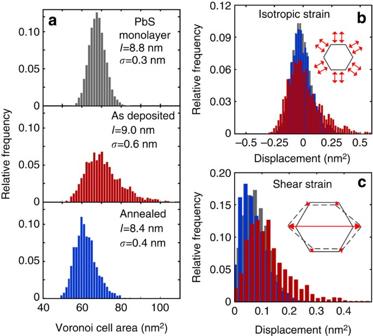Figure 3: Effect of solvent annealing on the strain for an epitaxial assembly withf=−6%. (a) Distribution of Voronoi cell areas for the PbS NC monolayer (grey) and Au NCs before (red) and after (blue) solvent annealing forf=−6%. Histograms of the measured (b) isotropic and (c) shear strain before (red) and after (blue) solvent annealing compared with that for the underlying PbS NC monolayer (grey). Insets are schematics of the strain modes. Figure 3: Effect of solvent annealing on the strain for an epitaxial assembly with f =−6%. ( a ) Distribution of Voronoi cell areas for the PbS NC monolayer (grey) and Au NCs before (red) and after (blue) solvent annealing for f =−6%. Histograms of the measured ( b ) isotropic and ( c ) shear strain before (red) and after (blue) solvent annealing compared with that for the underlying PbS NC monolayer (grey). Insets are schematics of the strain modes. Full size image Sub-monolayer epitaxy It is important to understand whether the kinetics of NC island nucleation and growth are similar to those observed in atomic epitaxy. The growth of non-strained atomic islands obeys a scaling law of the form n s ( θ )= θS −2 ξ ( s / S ), s ≥2, where s is the size (number of NCs) of the individual islands, n s ( θ ) is the density of islands of size s at coverage θ , S is the average island size given by S =∑ s ≥2 sn s ( θ )/∑ s ≥2 n s ( θ ), and ξ ( s/S ) is the scaling function which is coverage-independent [20] , [21] . 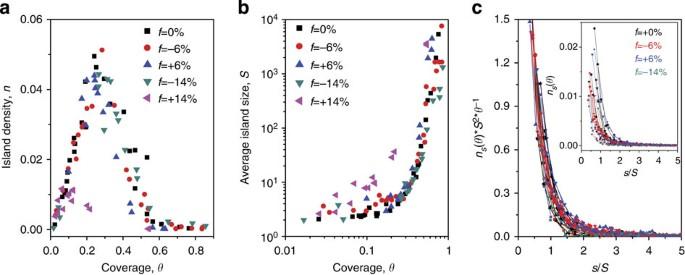Figure 4: Island statistics in the sub-monolayer regime. (a) Plot of the island densitynand (b) average island sizeSat different coverageθfor different lattice misfits after solvent annealing. (c) Scaled island size distribution curves for different lattice misfits at multiple coverages,θ<0.2. The inset shows the unscaled island size distribution; additional examples are given inSupplementary Fig. 8. Island is defined as a cluster of two or more NCs. Figure 4a,b shows island density n (number of islands per available landing site in the substrate monolayer) and S obtained for different lattice misfits as a function of θ . One striking observation is that all n and S distribution curves, except those for f =+14%, follow the same trend, with n peaking at θ ~0.25 and approaching percolation ( n →0; S →∞) at θ ~0.55. Furthermore, the experimental n s ( θ ) data for f =+6%, 0, −6% and −14% at θ ≤0.2 all collapse onto a common scaling function ξ ( s/S ) as shown in Fig. 4c and Supplementary Fig. 8 . The shape of ξ ( s/S ) is similar to that predicted by Monte Carlo simulations of post deposition island scaling behaviour with a critical island size i =1 (NC dimers act as smallest stable islands) and f =0% (ref. 22 ). In contrast, for the case of f =+14%, where Au NCs align poorly with the substrate ( Fig. 2c ), formation of stable, immobile islands requires more than two NCs ( i >1) ( Fig. 4b ). This difference is highlighted through snapshots at θ ~0.2 to 0.25 for f =+14%, 0% and −14% as shown in Supplementary Fig. 9 . The increase of the critical island size at large positive misfit accounts for the lower n and larger S values in Fig. 4a,b , respectively [18] , [22] . These results show that the island size distribution and growth dynamics in NC epitaxy are captured by the scaling theory commonly used to model atomic homoepitaxy [2] , [22] . The invariance of island dynamics across a broad range of lattice misfits is not typical for strained atomic epitaxy; however, this may be a generic feature of ‘soft’ epitaxy, where NCs and other soft objects can tolerate significant strain compared with their atomic counterparts due to shallow interparticle potentials. Figure 4: Island statistics in the sub-monolayer regime. ( a ) Plot of the island density n and ( b ) average island size S at different coverage θ for different lattice misfits after solvent annealing. ( c ) Scaled island size distribution curves for different lattice misfits at multiple coverages, θ <0.2. The inset shows the unscaled island size distribution; additional examples are given in Supplementary Fig. 8 . Island is defined as a cluster of two or more NCs. Full size image To further demonstrate the exceptional strain tolerance of ‘soft’ NC epitaxy, we use a periodically curved substrate with local variations of lattice spacing, formed by ‘draping’ monolayers of PbS NCs (8.3 and 8.8 nm) over a layer of 230 nm polystyrene (PS) beads as shown in Fig. 5a and Supplementary Fig. 10 . The conformation of the NCs monolayers to the PS colloids results in a substrate with complex curvature and non-uniform strain distribution; however, the NCs monolayers still control the epitaxial growth of the 8.3 nm Au NC adlayer ( Fig. 5 ). At θ ~0.2, the strain distribution in the draped NC monolayer results in the spatial patterning of the Au NC adlayer near the regions with zero-curvature ( Fig. 5b ). As θ approaches ~0.7–0.8, the formation of a uniform adlayer similar to that observed on a flat substrate is observed ( Fig. 5c ). Due to the softness of the interparticle potentials, minimal disruption in the epitaxial assembly is observed as compared with assembly on a planar surface ( Supplementary Figs 11 and 12 ). These results suggest that the softness of the interparticle potential enables the coherent formation of epitaxial adlayers over a wide range of lattice misfits and surface curvatures. 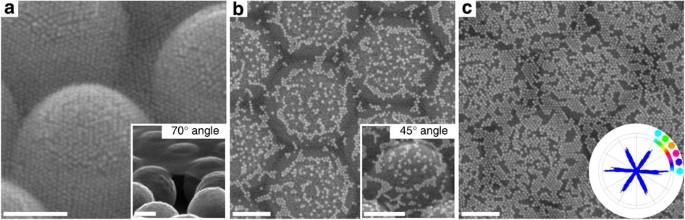Figure 5: Epitaxy on non-planar NC superlattices. (a) SEM image of a monolayer of 8.8 nm PbS NCs draped over hexagonally packed 230 nm polystyrene (PS) beads. Inset: SEM image showing the suspended monolayer viewed at a 70° angle. (b,c) SEM images of 8.3 nm Au NCs assembled on a monolayer of 8.8 nm PbS NCs draped over 230 nm PS colloids at (b)θ~0.2 and (c)θ~0.8. Inset inbis an SEM image of the assembly viewed at a 45° angle. Inset incshows the bond angle plot for the epitaxial NC adlayer. All scale bars, 100 nm. Figure 5: Epitaxy on non-planar NC superlattices. ( a ) SEM image of a monolayer of 8.8 nm PbS NCs draped over hexagonally packed 230 nm polystyrene (PS) beads. Inset: SEM image showing the suspended monolayer viewed at a 70° angle. ( b , c ) SEM images of 8.3 nm Au NCs assembled on a monolayer of 8.8 nm PbS NCs draped over 230 nm PS colloids at ( b ) θ ~0.2 and ( c ) θ ~0.8. Inset in b is an SEM image of the assembly viewed at a 45° angle. Inset in c shows the bond angle plot for the epitaxial NC adlayer. All scale bars, 100 nm. Full size image Surface reconstructions When the lattice misfit falls in a specific range, the interface between two crystal lattices can adopt non-trivial registry patterns, known as surface reconstructions. For example, when 8.3 nm Au NCs are deposited on 14.0 nm PbS NC monolayers ( f ~−40%) the epitaxial adlayer shows six Au NCs surrounding each large PbS NC ( Fig. 6a ). Following the Wood’s notation, we can describe this interface as a (1/√3 × 1/√3)R30° surface reconstruction, where the Au NC adlayer forms a hexagonal lattice with b=a /√3, rotated by 30° with respect to the substrate lattice. Such a reconstruction is expected since f ~−40% is very close to 1/√3 lattice contraction. The increase of coverage by depositing more Au NCs at such extreme f -value results in the formation of three-dimensional superlattices with hexagonally packed layers rotated by 30° with respect to the underlying PbS NC monolayer ( Supplementary Fig. 13 ), highlighting the ability to assemble a coherent interface even at very large misfit. 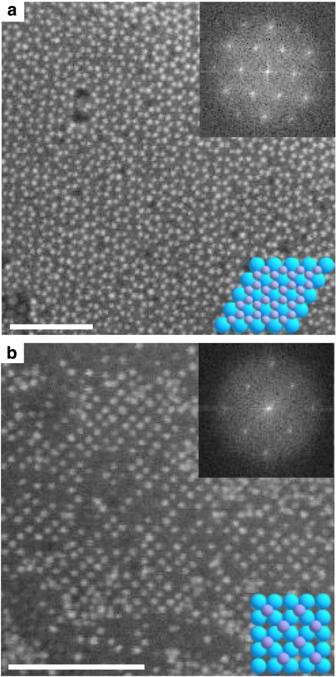Figure 6: Lattice reconstructions in the epitaxial NC adlayer. (a) SEM image showing the (1/√3 × 1/√3)R30° surface reconstruction of Au NC adlayer on top of a hexagonally packed PbS NC monolayer atf=−40% (8.3 nm Au NCs over 14.0 nm PbS NCs) where the Au NC lattice is rotated 30° with respect to the PbS NC monolayer. (b) SEM image of the (√2 × √2)R45° surface reconstruction of Au NCs on the NC superlattice substrate with square arrangement of PbS NCs atf=−6%. Lower insets are structural models of how the deposited NCs (purple) assemble on the PbS NC monolayer (blue). Upper insets are FFTs highlighting the long-range hexagonal order of the Au NCs. All scale bars, 100 nm. Figure 6: Lattice reconstructions in the epitaxial NC adlayer. ( a ) SEM image showing the (1/√3 × 1/ √ 3)R30° surface reconstruction of Au NC adlayer on top of a hexagonally packed PbS NC monolayer at f =−40% (8.3 nm Au NCs over 14.0 nm PbS NCs) where the Au NC lattice is rotated 30° with respect to the PbS NC monolayer. ( b ) SEM image of the (√2 × √2)R45° surface reconstruction of Au NCs on the NC superlattice substrate with square arrangement of PbS NCs at f =−6%. Lower insets are structural models of how the deposited NCs (purple) assemble on the PbS NC monolayer (blue). Upper insets are FFTs highlighting the long-range hexagonal order of the Au NCs. All scale bars, 100 nm. Full size image To further explore the extent to which NCs can assemble on surfaces, we studied epitaxial growth as a function of surface facets. A unique surface reconstruction is observed at f =−6% on the NC superlattice substrate with square NC packing, where Au NCs form a non-close packed layer with (√2 × √ 2)R45° surface reconstruction over the PbS NCs template. This result indicates that NC adlayers have the ability to reconstruct the surface with different structures and packing densities. Transition from first to second epitaxial layer The three major modes of epitaxial growth include: Volmer–Weber or island growth; Frank van der Merwe or layer-by-layer growth; and Stranski–Krastanov (SK) or layer-than-island growth ( Supplementary Fig. 14 ). The different growth modes are influenced by the degree of lattice misfit between the layers, as well as, the interaction energies between NCs in the deposit and substrate layers [2] . Lattice misfit is studied by depositing Au NCs on various size PbS NC monolayers, while the effect of interaction energies is examined by varying the composition of the deposited NCs at a fixed lattice misfit. We examined these effects as a function of coverage density and solvent annealing. For Au NCs on PbS NCs monolayers, the island density plot ( Fig. 4a ) shows that at θ ~0.55 the islands of Au NCs percolate into a continuous network ( Supplementary Fig. 15 ). As coverage increases towards a nearly complete adlayer, the transition from sub-monolayer to three-dimensional growth begins with the nucleation of a second NC adlayer ( Fig. 7 ). The difference in SEM contrast between the first and second Au NC adlayers is sufficient to apply particle tracking and measure bond angle distributions selectively for NC in each layer ( Supplementary Fig. 16 ). Such analysis reveals important trends in the alignment of the first and second adlayers. In the cases of large lattice misfit ( f =±14%), the as-deposited adlayers are poorly aligned and there is minimal difference in organization of the first and second layers due to the high degree of strain ( Fig. 7a,i ). At f =−14%, the tensile strain allows both layers to relax after solvent annealing, while at f =+14%, the compressive strain prevents significant relaxation ( Fig. 7b,j ). However, for the as-deposited samples at smaller misfits, −6%≤ f ≤+6%, the wetting layer aligns with the substrate while the second layer is highly disordered. After solvent annealing, an increased sharpness of the bond angle plots for both layers is observed ( Fig. 7 ). Notably, the standard deviation (s.d.) of the bond angle plots decreases by 40–60% for the second layer, whereas for the wetting layer the s.d. typically decreases by 5–10%, indicating that the improvement in alignment is much greater for the second layer. In addition, at all lattice misfits tested, the second layer exhibits reduced angular dispersion compared with the wetting layer ( Supplementary Table 3 ), likely because of additional strain relaxation in the second adlayer. 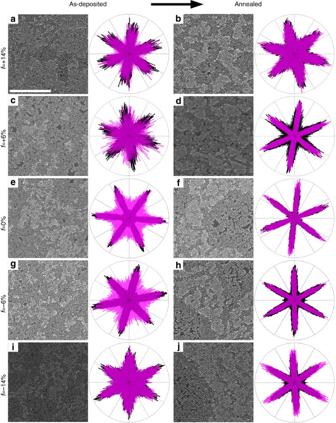Figure 7: Characterization of Au NC organization in the first and second adlayers at 1<θ<2. SEM images of epitaxial assemblies at 1<θ<2 at (a,b)f=+14%, (c,d)f=+6%, (e,f)f=0%, (g,h) 8f=−6% and (i,j)f=−14% before (a,c,e,g,i) and after (b,d,f,h,j) solvent annealing. Bond angle plots for each image show the orientation of all bonds in the top (pink) and bottom (black) layers. The orientation of the bonds in the different adlayers were analyzed independently. Scale bar, 200 nm. Figure 7: Characterization of Au NC organization in the first and second adlayers at 1< θ <2. SEM images of epitaxial assemblies at 1< θ <2 at ( a , b ) f =+14%, ( c , d ) f =+6%, ( e , f ) f =0%, ( g , h ) 8 f =−6% and ( i , j ) f= −14% before ( a , c , e , g , i ) and after ( b , d , f , h , j ) solvent annealing. Bond angle plots for each image show the orientation of all bonds in the top (pink) and bottom (black) layers. The orientation of the bonds in the different adlayers were analyzed independently. Scale bar, 200 nm. Full size image Our results suggest a kinetic bottleneck in the epitaxial growth of the second NC adlayer, which indicates the general importance of solvent annealing during multilayer NC epitaxy. We are not aware of similar effects in atomic epitaxy. Such a kinetic bottleneck may originate from the difference in critical island size for the first and second NC adlayers [18] . In the first adlayer, the assembly of Au NCs occurs on top of the layer of PbS NCs while the second adlayer of Au NCs forms on top of the initial Au NC adlayer. The difference in the Hamaker constants for PbS and Au results in the strength of each ‘bond’ formed between adlayer NCs and the underlying substrate to be greater in the second NC adlayer than in the first adlayer ( Supplementary Discussion and Supplementary Fig. 17 ). Correspondingly, the activation energy for diffusion of Au NCs in the second adlayer is higher compared with that for the first adlayer. As a result of the inhibited diffusion of Au NCs in the second adlayer, the critical island size may reduce to i =0 for the second adlayer at room temperature. A long-range ordered layer cannot assemble on a hexagonal lattice with i =0 because the number of ‘landing’ sites is twice the number of NCs that can be landed (it is, in fact, the origin of fcc and hcp polymorphs). Therefore, when i =0, a disordered second adlayer forms. Solvent annealing at an elevated temperature facilitates NC diffusion and increases i from 0 to 1, which results in a well-ordered monolayer ( Fig. 7 ). Three-dimensional epitaxial growth As the coverage increases to θ >2, discrete islands form on top of a few wetting layers of Au NCs ( Fig. 8a,c ). The size and concentration of the islands increases with increasing lattice misfit ( Supplementary Fig. 18 ). This film morphology resembles that of SK growth in which islands grow on top of one or several coherent adlayers [2] ; however, it can also be a transient state caused by rapid evaporation of the carrier solvent. To resolve this ambiguity, we solvent anneal the assemblies. In the cases where f =0 and −6%, annealing results in the complete disappearance of islands yielding smooth, layered superlattices ( Supplementary Fig. 19 and Fig. 8d , respectively). At f =0%, the adlayers are smooth and unstrained ( Supplementary Fig. 20 ), while at f =−6%, a triangular mesh of misfit dislocations form to relax lattice misfit ( Fig. 8b ) [23] . This strain relaxation is also evident from the gradual decrease of the Voronoi cell area as θ increases from monolayer to multilayer for f =−6% ( Fig. 8e ). These observations suggest that at f =0% and −6% island formation is not thermodynamically favourable. A similar behaviour is observed at f =+6%. However, in addition to smooth, layer-by-layer growth, layer-then-island growth is also observed ( Supplementary Fig. 21 ). 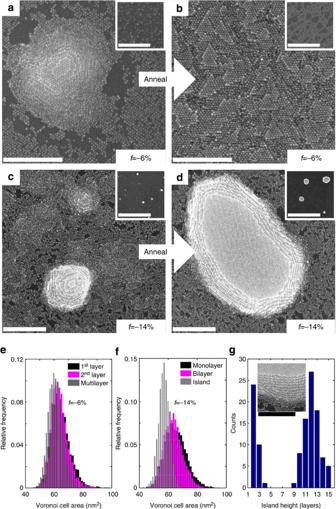Figure 8: Multilayer epitaxial growth. (a,b) SEM images of epitaxial assemblies atf=−6% atθ>2 for (a) before and (b) after solvent annealing show the disappearance of islands. (c,d) SEM images of epitaxial assemblies atf=−14% atθ>2 (c) before and (d) after solvent annealing reveal the formation of Stranski–Krastanov islands. Insets ina–dare low magnification SEM images. (e,f) Distribution of Voronoi cell areas for Au NCs in different layers: forf=−6%, multilayer is a 3–5 monolayer film, while forf=−14%, the island is the top layer of a 12 monolayer thick island. (g) Distribution of the island heights observed atf=−14% after solvent annealing. The inset is an SEM image at a 20° tilt of an Au NC island. All scale bars are 200 nm except for those insets ina–d. The scale bars for insets ina–dare 5 μm. Figure 8: Multilayer epitaxial growth. ( a , b ) SEM images of epitaxial assemblies at f =−6% at θ >2 for ( a ) before and ( b ) after solvent annealing show the disappearance of islands. ( c , d ) SEM images of epitaxial assemblies at f =−14% at θ >2 ( c ) before and ( d ) after solvent annealing reveal the formation of Stranski–Krastanov islands. Insets in a – d are low magnification SEM images. ( e , f ) Distribution of Voronoi cell areas for Au NCs in different layers: for f =−6%, multilayer is a 3–5 monolayer film, while for f =−14%, the island is the top layer of a 12 monolayer thick island. ( g ) Distribution of the island heights observed at f =−14% after solvent annealing. The inset is an SEM image at a 20° tilt of an Au NC island. All scale bars are 200 nm except for those insets in a – d . The scale bars for insets in a – d are 5 μm. Full size image When the lattice misfit increased to f =−14%, solvent annealing results in a very different final structure. As deposited, the Au NCs form poorly ordered adlayers with small islands of varying size ( Fig. 8c ). Solvent annealing transforms the epitaxial assembly into large (>0.5 μm in diameter) islands with flat tops over a monolayer thick wetting layer of Au NCs ( Fig. 8d ). Both the wetting layer and islands are aligned with the substrate providing a first example of NC SK epitaxy ( Supplementary Figs 22 and 23 ). Inside the islands, strain is released by coherent lattice contraction as indicated by the reduction in Voronoi cell areas ( Fig. 8f and Supplementary Fig. 22c ) [2] , [24] . While some islands possess defect free layers ( Fig. 8d ), many contain screw dislocations ( Supplementary Fig. 24 ) [2] , [25] . However, all islands show a uniform height of ~12 monolayers ( Fig. 8g ). Although areas with two or three adlayers are occasionally found, no islands thinner than nine monolayers are observed, indicating a window of ‘forbidden’ island heights. Similar island height distributions are observed after 2 and 18 h of solvent annealing ( Supplementary Fig. 25 ). This observation supports the thermodynamic rather than the kinetic nature of such a counter intuitive height distribution. A similar phenomenon has been observed in atomic metal on semiconductor systems, such as Ag and Pb on Si, and was originally attributed to electronic quantum size effects [26] , [27] , [28] . Later, Prieto and Markov [28] proposed that the absence of thin SK islands is caused by the interplay of strain and edge energies in coherent epitaxial islands, where a minimum height is needed to relieve strain from lattice misfit. We consider the latter scenario more plausible for NC epitaxy. Interestingly, both before and after solvent annealing, the Au NCs islands are aligned with the substrate; however, a consistent slight rotation (~5°) of the island tops with respect to the substrate is observed ( Supplementary Figs 22,23,26 ). The small rotation of epitaxial islands helps reduce the interfacial strain. It has been observed in atomic systems as discussed in ref. 3 . Epitaxy of Non-spherical NCs NCs further provide the opportunity to study the role of shape in epitaxy. Non-spherical objects are of particular importance for soft matter as molecular, bio, nano and mesoscale species rarely adopt spherical shapes. As a first example of the influence of shape on epitaxial growth, we deposit 55 × 8 nm CdSe nanorods (NRs) on smooth and periodic substrates ( Fig. 9 ). On a smooth substrate, NRs assemble into a smectic (Sm) phase ( Fig. 9a ), consistent with the previous studies [29] . However, when deposited on a hexagonal-packed PbS NC monolayer, the substrate templates the assembly along one of the three equivalent directions ( Supplementary Fig. 24 ). At sub-monolayer coverage, NRs form collections of small domains, unidirectionally aligned with the underlying lattice ( Fig. 9b,c ). At higher coverage, the growth of Sm domains, which were observed on smooth substrates, is suppressed ( Fig. 9d ). This indicates that for NRs, the periodic potential of the substrate has a poisoning effect on the organization of the adlayer, in contrast to the epitaxy of spherical NCs, where an ordered substrate induces order in the adlayer. Of note, line defects in the substrate, like ripples in a PbS NC monolayer, act as nucleation centres for the epitaxial Sm phase ( Fig. 9e and Supplementary Fig. 28 ). At 1< θ , wrinkles result in an increase in the domain size of the unidirectional NRs, which transition into Sm assemblies of NRs at θ >1 ( Supplementary Fig. 28 ). 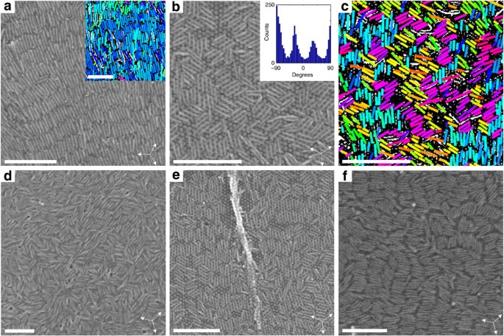Figure 9: Epitaxy of CdSe nanorods on PbS NC superlattices. SEM images of CdSe nanorods (55 nm long and 8 nm in diameter) on (a) a flat surface and (b) a 12 nm PbS NC monolayer atθ<1. Colour coded images ofa,bare given in the inset ofaand panelcin which the nanorods are coloured according to orientation. Inset tob: plot of the angular distribution of the nanorods inb. SEM images of CdSe NRs atθ~1 on a (d) smooth and (e) wrinkled 12 nm PbS NC monolayer. (f) SEM image of 8 nm diameter CdSe NRs on a monolayer of 7.3 nm PbS NCs atθ~1. The arrows in the bottom right corners give the orientation of the underlying PbS NC monolayers. All scale bars, 200 nm. Figure 9: Epitaxy of CdSe nanorods on PbS NC superlattices. SEM images of CdSe nanorods (55 nm long and 8 nm in diameter) on ( a ) a flat surface and ( b ) a 12 nm PbS NC monolayer at θ <1. Colour coded images of a , b are given in the inset of a and panel c in which the nanorods are coloured according to orientation. Inset to b : plot of the angular distribution of the nanorods in b . SEM images of CdSe NRs at θ ~1 on a ( d ) smooth and ( e ) wrinkled 12 nm PbS NC monolayer. ( f ) SEM image of 8 nm diameter CdSe NRs on a monolayer of 7.3 nm PbS NCs at θ ~1. The arrows in the bottom right corners give the orientation of the underlying PbS NC monolayers. All scale bars, 200 nm. Full size image Similar to spherical NCs, lattice misfit plays a role on the epitaxy of NRs. We observe that the NRs are able to align with the substrate when the diameter of the NR is less than the lattice parameter of the NC template ( f ′= (b ′ −a)/a <0, where b ′ is the diameter of the NR) as seen in Fig. 9b,d,e and Supplementary Figs 29a and 30 . However, when f ′>0, poor alignment is observed ( Fig. 9f and Supplementary Fig. 29b ) and large Sm domains form. The effect of lattice misfit is noticeable at θ ~1, where different structures are observed. For the case where f ′ <0, a jammed phase with small ordered domains is observed ( Fig. 9d ), while when f ′>0, rather large Sm domains form ( Fig. 9f ). In the latter case, the directors of the NR Sm assemblies do not align with the substrate lattice. In addition, we observe that NR assembly is affected by the relative NR length. By comparing the epitaxial assembly at f ′=−9%, an improvement in alignment is observed as the ratio of NR length to NC diameter increases ( Supplementary Figs 29a and 30 ). These results illustrate that the quality of NR epitaxial assembly is influenced by both the length and the width of the NRs. Epitaxy on binary NC superlattices In this section, we show that NC epitaxy can occur on the surface of more complex NC superlattices. In addition to hexagonally packed NC monolayers, NCs can self-assemble into complex binary and ternary superlattices [10] , [11] . Recently, methods were developed to assemble thin, binary NC membranes [30] . Using these methods, we assemble superlattices composed of 15.5 nm Fe 3 O 4 and 6.0 or 8.3 nm Au NCs with various packing structures (AlB 2 , CaB 6 and bcc-AB 6 isostructural with Cs 6 C 60 ). These membranes are then used as substrates for the epitaxial assembly of Au and PbS NCs ( Fig. 10 and Supplementary Figs 31 and 32 ). Epitaxial assembly is first investigated by depositing 8.3 nm Au NCs on these membranes, where ordered domains over several hundreds of nanometers are observed. We find that Au NCs reconstruct the surface by assembling in the interstitial sites between the Fe 3 O 4 NCs ( Fig. 10b,d ). The NCs alignment with the substrate is seen by comparing FFTs, where the symmetry of the binary membrane is retained in the epitaxial assembly. 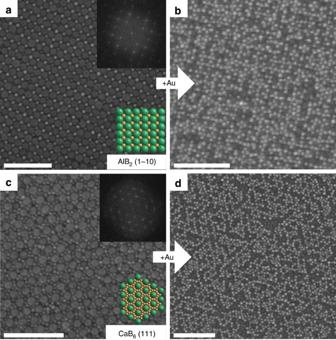Figure 10: Epitaxial assembly of Au NCs on binary NC superlattices. (a) SEM image of the 1–10 projection of the AlB2structure assembled from 15.5 nm Fe3O4and 8.3 nm Au NCs. (b) SEM image of the epitaxial assembly formed by the deposition of 8.3 nm Au NCs on the structure ina. (c) SEM image of the 111 projection of the CaB6structure assembled from 15.5 nm Fe3O4and 6.0 nm Au NCs. (d) SEM image of the epitaxial assembly formed by the deposition of 8.3 nm Au NCs on the structure inc. Upper insets ina,care FFTs of the images. Lower insets ina,care models of the lattice projections. All scale bars, 100 nm. Figure 10: Epitaxial assembly of Au NCs on binary NC superlattices. ( a ) SEM image of the 1–10 projection of the AlB 2 structure assembled from 15.5 nm Fe 3 O 4 and 8.3 nm Au NCs. ( b ) SEM image of the epitaxial assembly formed by the deposition of 8.3 nm Au NCs on the structure in a . ( c ) SEM image of the 111 projection of the CaB 6 structure assembled from 15.5 nm Fe 3 O 4 and 6.0 nm Au NCs. ( d ) SEM image of the epitaxial assembly formed by the deposition of 8.3 nm Au NCs on the structure in c . Upper insets in a , c are FFTs of the images. Lower insets in a , c are models of the lattice projections. All scale bars, 100 nm. Full size image Next, we investigate the assembly of 14 nm PbS NCs on these membranes ( Supplementary Fig. 32 ). We find that PbS NCs assemble according to the symmetry of the Fe 3 O 4 NC lattice, resulting in either a square or hexagonal structure. In this case, a single PbS NC sits over the interstial site between Fe 3 O 4 NCs. These results are significant because the ability of binary NC superlattices to control the epitaxial assembly of both large and small NCs creates a potential path to generate more complex NC interfaces. These examples of spherical NCs and NRs show that epitaxial assembly on a periodic substrate can either promote ordering of the adlayer (for spherical NCs) or suppress the growth of ordered domains (for NRs). In the former case, epitaxy and solvent annealing provide a route for the formation of coherent interfaces with an impressive tolerance to lattice misfit. In the latter case, insights into the challenges present for the formation of epitaxial NC superlattices are revealed. NC epitaxy may offer new avenues to generate more complex NCs interfaces as seen through the ability to form coherent interfaces under high levels of strain, at extreme lattice misfit and on complex surface topologies. Through the formation of the complex interfaces, NC self-assembly provides the ability to study phenomena that are unique to the ‘soft’ materials world. The degree of NC ‘softness’ can be varied by changing ligands. Shorter ligands create stiffer interactions while longer ligands are more flexible. In addition, tailoring surface chemistry to direct epitaxy of nanoscale objects would be another exciting direction for future studies. The next step is applying these techniques to the fabrication of NC-based devices, whose function is directly influenced by the perfection of the interface. NC synthesis Highly monodisperse Au, CdSe, Fe 3 O 4 and PbS NCs and CdSe NRs were synthesized according to literature methods. Additional details are provided in the Supplementary Methods . In brief, oleate-capped PbS NCs were synthesized by reacting lead oleate with bis(trimethylsilyl)sulphide in a solution of oleic acid and octadecene. Their size was tuned by varying the ratio of precursors. Dodecanethiol-capped Au nanoparticles were synthesized by the reduction of HAu(PPh 3 ) in benzene with borane- t -butylamine complex at 80 °C. Self-assembly of NC monolayers PbS NC monolayers were self-assembled based on literature techniques [17] at the air–liquid interface, as shown in Supplementary Fig. 33 . In a typical process, 40 μl of a NC solution in toluene (~0.5 mg ml −1 ) was deposited over a 100 μl droplet of deionized water on a glass slide. The toluene was allowed to fully evaporate for ~20 min before the monolayer was transferred to a 1 × 1 cm 2 silicon wafer by stamping the surface of the water droplet. Excess water was carefully removed with filter paper. The NC monolayers were allowed to dry in air for ~1 week before use and then rinsed with ethanol and dried under nitrogen flow. Formation of polystyrene colloid monolayers Silicon wafers (1 × 1 cm 2 ) were treated with oxygen plasma (15 min) to become hydrophilic. A 10 μl drop of 230 nm polystyrene (PS) colloids in MilliQ water was deposited on the Si wafer and allowed to dry (~1 h). To image the samples in SEM, the PS monolayers were sputter coated with an 8.0-nm-thick layer of Pt/Pd using a Ted Pella 208HR High Resolution Sputter Coater Formation of curved PbS NCs monolayers A scheme depicting the assembly of curved PbS NCs monolayers is shown in Supplementary Fig. 34 . In brief, the PS-coated Si wafer assembled above was cut into four equal squares (0.5 × 0.5 cm 2 ) and placed on a glass slide covered with Teflon tape. Deionized water (~30 μl) was deposited on the PS/Si covering the entire Si wafer. Then, two drops of a colloidal solution of PbS NCs in toluene (0.5 mg ml −1 ) from a 100 μl pipette tip were placed over the droplet of water on each Si wafer piece. The water and PbS solution were then allowed to dry on top of the PS-coated Si wafer for 1.5 h, resulting in the formation of a PbS NC monolayer draped over the PS colloid monolayer. Assembly of binary NC superlattices Binary NC superlattices were assembled according to the procedure developed by Dong, et al . [30] In brief, the ratio between Fe 3 O 4 and Au NC was tuned through solvent evaporation self-assembly until the desired structures were formed. Using this NC ratio, binary membranes were assembled. A 1.5-cm-wide by 0.5-cm-deep square well was made in a Teflon block. A substrate (Si wafer or transmission electron microscopy grid) was placed at the bottom of the well and covered with a layer of diethylene glycol (~0.3 mm deep). Twenty microlitres of a binary mixture of Fe 3 O 4 and Au NCs in hexane were added to the edge of the well. The well was covered with a glass cover slide and the hexane was allowed to evaporate. Once dry, the diethylene glycol was removed via syringe, leaving the self-assembled membranes on the substrates. The substrates were then dried under vacuum for ~24 h before use. Formation of epitaxial assemblies PbS NC monolayers, binary membranes and curved PbS monolayer assemblies were used as substrates for the epitaxial assembly. The epitaxial NCs (Au, Fe 3 O 4 , PbS and CdS NRs) were dried and redispersed in a mixture of 9:1 hexane:octane by volume and then drop cast onto the NC monolayer substrates ( Fig. 1 ). To vary the concentration of NCs, the stock NC solution was diluted with pure solvent. For each experiment, two samples were prepared and one was characterized as deposited while the other was solvent annealed. The samples were solvent annealed in a preheated 40 °C oven (Yamato ADP310C vacuum oven) in a recrystallization dish on a Teflon stand surrounded by toluene. The dish was covered with a piece of watch glass, as shown in Supplementary Fig. 35 . NC assemblies were solvent annealed for 15 min to 20 h, although the majority of the samples were solvent annealed for 2 h. Assembly of macroscopic NC superlattices Phase diffusion self-assembly was carried out according to literature procedures [31] . In brief, the crystallization of CdSe and PbS NCs was carried out through a two-layer phase diffusion technique in vertically positioned glass test tubes. In a typical experiment, a 0.8 cm inner diameter tube was filled with 1.2 ml of a colloidal solution of CdSe and PbS NCs in toluene. The ratio of CdSe/PbS was varied from 1:1 to 10:1 by mole while keeping the total concentration <1 mg ml −1 . A layer of ethanol (1.5 ml) was carefully added to the tube which was subsequently capped and left in the dark for ~1 week. During this time, the NC superlattices nucleated and grew on walls of the tube and on the thin silicon substrate positioned vertically in the tube. After completion of the experiment, the solvent was carefully removed and the silicon substrate was taken out of the tube and rinsed with acetone. The superlattices were studied by optical microscopy and SEM. Characterization AFM images of PbS NC monolayers were taken on a Veeco/Bruker Multimode 8 in tapping mode. SEM images of the NC assemblies were collected on a FEI NanoSEM 200 equipped with a GV10 Asher, plasma cleaner manufactured by Ibss Group, Inc. Imaging was carried out with an accelerating voltage of 10 to 20 kV at a working distance between 4.0 and 5.5 mm. Transmission electron microscopy imaging was performed using an FEI Tecnai F30 microscope operated at an accelerating voltage of 300 kV. Optical microscopy images were taken on an Olympus BX51 microscope. Absorption spectra of the colloidal PbS NC solutions were collected with an Agilent Cary 5000 UV-vis-NIR spectrophotometer. Particle tracking analysis Particle tracking of the SEM images was performed using the methods developed by Crocker and Grier [19] . Home-written MatLab codes were used. Particle tracking was carried out on SEM images with horizontal field widths of 0.75–1.5 μm and vertical field heights of 0.6–1.3 μm, resulting in images with ~1–3 × 10 5 PbS NCs in the substrate layer. The coverage varied with the number of deposited Au NCs and was calculated as the number of Au NCs per sites in the substrate layer. Statistical analysis of NC diameter and strain was carried out on images with 10 4 –10 5 NCs. While the average resolution of the raw images was ~1.2 nm per pixel, sub-nanometer accuracy was possible in locating centres of individual NCs. For all reported data, a minimum of two similar images were analyzed for reproducibility. A scheme depicting the process is shown in Supplementary Fig. 36 with an analyzed bond angle plot in Supplementary Fig. 37 . Additional details describing the process are provided in Supplementary Note 3 . How to cite this article: Rupich, S. M. et al . Soft epitaxy of nanocrystal superlattices. Nat. Commun. 5:5045 doi: 10.1038/ncomms6045 (2014).